Mutations in epigenetic regulators including SETD2 are gained during relapse in paediatric acute lymphoblastic leukaemia Relapsed paediatric acute lymphoblastic leukaemia (ALL) has high rates of treatment failure. Epigenetic regulators have been proposed as modulators of chemoresistance, here, we sequence genes encoding epigenetic regulators in matched diagnosis–remission–relapse ALL samples. We find significant enrichment of mutations in epigenetic regulators at relapse with recurrent somatic mutations in SETD2 , CREBBP , MSH6 , KDM6A and MLL2 , mutations in signalling factors are not enriched. Somatic alterations in SETD2, including frameshift and nonsense mutations, are present at 12% in a large de novo ALL patient cohort. We conclude that the enrichment of mutations in epigenetic regulators at relapse is consistent with a role in mediating therapy resistance. Relapse occurs in 15–20% of paediatric ALL and 50% of adult ALL patients. Compared to de novo leukaemia, relapsed leukaemia is chemoresistant and long-term survival is poor; however, the genetic basis for this is not well understood. Studies of matched diagnosis and relapse ALL samples by SNP arrays demonstrated that 92% of relapsed ALL had DNA copy number variant (CNV) changes from diagnosis. Surprisingly, over half of relapses are missing CNVs present in the predominant clone at diagnosis and appear to have derived from a minor subclone in many cases [1] . Targeting alterations that are frequently gained at relapse is therefore a rational therapeutic strategy, as these lesions are likely associated with chemotherapy resistance and clonal survival. Unfortunately, most CNV alterations gained at ALL relapse are difficult to target, such as CDKN2A or ETV6 deletion. Alterations in epigenetic regulators have recently been identified in genome and exome sequencing studies of chemotherapy resistant, very high-risk subsets of de novo ALL. For example, 48% of early T-cell precursor (ETP) ALL [2] and 60% of hypodiploid ALL [3] have somatic mutations in genes encoding epigenetic regulators. In addition, loss-of-function mutations in the histone acetyltransferase CREBBP have also been described in diagnostic samples from ALL patients who relapse, and in samples from relapsed patients [4] . As the enzymatic activities of CREBBP are directly opposed by histone deacetylases, this provided one possible rationale for why histone deacetylase inhibitors have activity in ALL. These studies suggest a broader paradigm in that mutations in epigenetic regulators may be associated with therapy resistance and can be targeted indirectly through inhibition of the enzymatic activity of opposing regulators. However, thus far, no published study has addressed the mutational frequency of epigenetic regulators at ALL relapse, and whether they are frequently enriched at relapse compared to at diagnosis. Here, we sequence matched sets of diagnosis–remission–relapse samples from paediatric ALL patients, and find a significant enrichment of mutations in epigenetic regulators at relapse, including the H3K36 trimethyltransferase SETD2. We conclude that these mutations are likely involved in chemotherapy resistance and deserve further study to define their role in the prognosis and treatment of ALL. 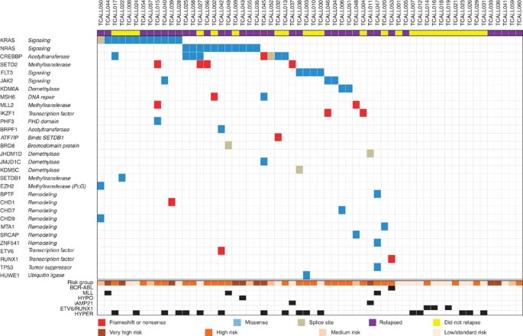Figure 1: Targeted hybrid capture sequencing identified somatic mutations in 70% of B-ALL patients. Matched tumour-remission samples from 60 paediatric B-ALLs were sequenced with targeted hybrid capture and somatic mutations in any tumour sample were identified. Genes on the left are organized by mutational frequency. The type of alteration is identified for each mutation as frameshift/stop, missense or splice site mutation. MLL, MLL rearranged; HYPO, hypodiploidy; iAMP21, intrachromosomal amplification of chromosome 21; HYPER, hyperdiploidy. Somatic mutations in epigenetic regulators in de novo ALL To study this, we performed custom exon-hybrid capture and Illumina sequencing of 472 known and putative epigenetic regulators and frequently mutated genes in leukaemia ( Supplementary Table 1 ) on matched diagnostic-remission samples from 60 paediatric B-ALL patients, and matched relapse samples from 30 of those patients that relapsed. 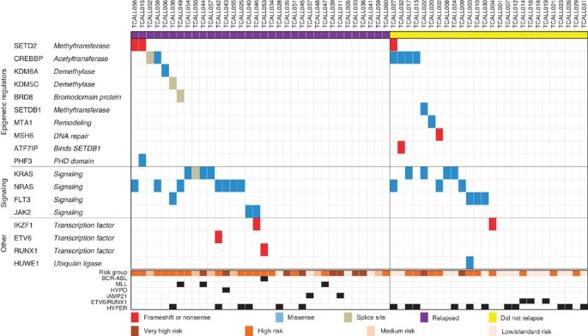Figure 2: Mutations in epigenetic regulators occur in 25% of B-ALL patients at diagnosis, including SETD2. Matched diagnosis and remission sample pairs from 60 paediatric B-ALL patients were baited with target hybrid capture, Illumina sequenced and somatic mutations were identified. Patients are organized by those that eventually relapsed (on the left), and those that did not (on the right). Final risk category and molecular subtypes listed below. MLL, MLL rearranged, HYPO, hypodiploidy, iAMP21, intrachromosomal amplification of chromosome 21, HYPER, hyperdiploidy. Patients in this cohort were those with paediatric ALL (primarily B cell), with a range of cytogenetics and risk groups ( Supplementary Table 2 ). In this cohort, relapsed patients had the bone marrow as a site of relapse, with over 60% marrow involvement. 70% of patients had an identified somatic mutation at diagnosis and/or relapse ( Fig. 1 ). Figure 1: Targeted hybrid capture sequencing identified somatic mutations in 70% of B-ALL patients. Matched tumour-remission samples from 60 paediatric B-ALLs were sequenced with targeted hybrid capture and somatic mutations in any tumour sample were identified. Genes on the left are organized by mutational frequency. The type of alteration is identified for each mutation as frameshift/stop, missense or splice site mutation. MLL, MLL rearranged; HYPO, hypodiploidy; iAMP21, intrachromosomal amplification of chromosome 21; HYPER, hyperdiploidy. Full size image Considering only samples from the time of diagnosis, somatic variants in epigenetic regulators were found in 25% of 60 B-ALL samples ( Fig. 2 ), which was similar to de novo T-ALL patients [5] . In contrast, 50% of B-ALL samples harboured a mutation in a signalling factor at diagnosis with recurrent mutations in the Ras pathway, including activating point mutations in KRAS and NRAS , which were often subclonal ( Supplementary Fig. 1A ). At diagnosis, recurrent mutations in epigenetic regulator genes were identified in CREBBP (10%) and SETD2 (5%). Figure 2: Mutations in epigenetic regulators occur in 25% of B-ALL patients at diagnosis, including SETD2. Matched diagnosis and remission sample pairs from 60 paediatric B-ALL patients were baited with target hybrid capture, Illumina sequenced and somatic mutations were identified. Patients are organized by those that eventually relapsed (on the left), and those that did not (on the right). Final risk category and molecular subtypes listed below. MLL, MLL rearranged, HYPO, hypodiploidy, iAMP21, intrachromosomal amplification of chromosome 21, HYPER, hyperdiploidy. Full size image SETD2 mutations in de novo ALL To more accurately determine the frequency of SETD2 mutations, which have not been previously described in B-ALL, the coding regions of SETD2 were PCR amplified and Illumina sequenced in a more representative, independent validation cohort of 125 de novo paediatric ALL patients. SETD2 mutations were found in 12% of the cohort and these leukaemias also frequently harboured mutations in the Ras pathway ( Fig. 3a ). Four patients harboured multiple SETD2 mutations. In total, we identified 24 SETD2 mutations in 19 out of 185 ALL patients, including seven loss-of-function frameshift or nonsense mutations, with no obvious hotspot mutations ( Fig. 3b ). 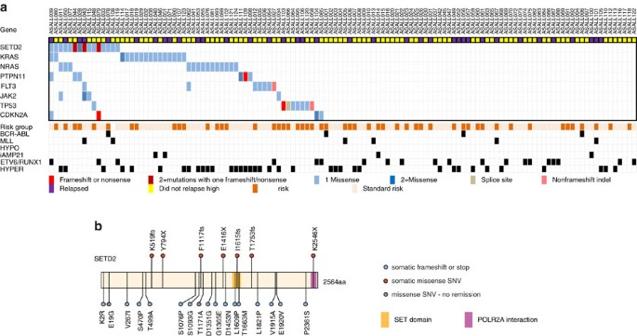Figure 3: SETD2 mutations inde novoALL. (a) Amplification and Illumina sequencing of coding exons of SETD2 and other frequently mutated genes in an validation cohort of 125de novoALL patients identified 20 additional SETD2 mutations in 15 patients (12%). Relapse status is noted above. Final risk category and molecular subtypes listed below. MLL, MLL rearranged; HYPO, hypodiploidy; iAMP21, intrachromosomal amplification of chromosome 21; HYPER, hyperdiploidy. (b) Schematic of somatic SETD2 mutations found in ALL patients. Altogether, SETD2 mutations were most prevalent in the MLL rearranged (22%) and ETV6-RUNX1 rearranged (13%) subtypes of ALL ( Supplementary Table 3 ). Of note, these two subtypes were underrepresented in the initial cohort, explaining the lower prevalence of SETD2 mutations in that cohort. Figure 3: SETD2 mutations in de novo ALL. ( a ) Amplification and Illumina sequencing of coding exons of SETD2 and other frequently mutated genes in an validation cohort of 125 de novo ALL patients identified 20 additional SETD2 mutations in 15 patients (12%). Relapse status is noted above. Final risk category and molecular subtypes listed below. MLL, MLL rearranged; HYPO, hypodiploidy; iAMP21, intrachromosomal amplification of chromosome 21; HYPER, hyperdiploidy. ( b ) Schematic of somatic SETD2 mutations found in ALL patients. Full size image Enrichment of mutations in epigenetic regulators at relapse Sequencing of the 30 matched relapsed samples showed a striking gain of mutations in epigenetic regulators, with 17 (57%) harbouring a mutation. Of the 11 patients that gained a mutation in an epigenetic regulator at the time of relapse, only 3 were detectable in a rare subclone at diagnosis. ( Fig. 4a ). As noted above, this frequency is comparable to other poor prognosis de novo ALL subgroups, such as hypodiploid and ETP ALL. In addition to the 11 gains, 5 patients retained the same mutations from diagnosis, and 1 patient had their clonal mutation reduced to a subclonal allele frequency at relapse ( Supplementary Fig. 1B ). Details of each identified somatic mutation in each patient and a summary of mutations by molecular subtype are available in the Supplementary Materials ( Supplementary Tables 3 and 4 ). 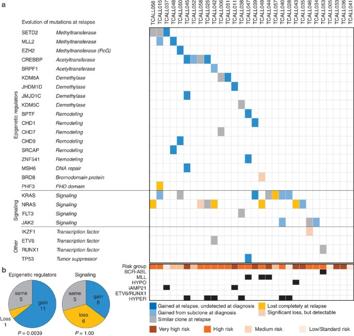Figure 4: Relapsed B-ALL is enriched for mutations in epigenetic regulators. (a) Gain or loss of somatic mutations in matched diagnosis-relapse samples from 30 paediatric B-ALL patients. Clonal mutations at relapse which were detected in a minor subclone at diagnosis and clonal mutations at diagnosis which became subclonal at relapse are shaded. MLL, MLL rearranged; HYPO, hypodiploidy; iAMP21, intrachromosomal amplification of chromosome 21; HYPER, hyperdiploidy. (b) Comparison of the number of patients which gain, lose or have the same number of mutations in epigenetic regulators and signalling factors at relapse. The McNemar test was used to calculate theP-values. Figure 4: Relapsed B-ALL is enriched for mutations in epigenetic regulators. ( a ) Gain or loss of somatic mutations in matched diagnosis-relapse samples from 30 paediatric B-ALL patients. Clonal mutations at relapse which were detected in a minor subclone at diagnosis and clonal mutations at diagnosis which became subclonal at relapse are shaded. MLL, MLL rearranged; HYPO, hypodiploidy; iAMP21, intrachromosomal amplification of chromosome 21; HYPER, hyperdiploidy. ( b ) Comparison of the number of patients which gain, lose or have the same number of mutations in epigenetic regulators and signalling factors at relapse. The McNemar test was used to calculate the P -values. Full size image By McNemar test, there was a statistically significant enrichment of the entire epigenetic group ( P =0.0039) ( Fig. 4b ) and SETD2 and CREBBP together ( P =0.045). In contrast, there was not a significant enrichment of somatic mutations in signalling factors such as NRAS , KRAS , FLT3 and JAK2 , as individual genes, or as a group. This was because there were as many patients gaining signalling mutations or mutational allele frequency as those losing them (six, McNemar test P =1.00) ( Fig. 4b ). The selective enrichment of epigenetic regulators is consistent with the hypothesis that mutations in genes encoding epigenetic regulators mediate chemotherapy resistance. Conversely, oncogenic mutations in signalling factors showed no enrichment, with frequent losses and gains, implying no direct role in modulating drug resistance and non-dependence on any particular mutation. Thus, solely targeting signalling factors by specific inhibition may not circumvent the development of chemoresistance. In total, recurrently mutated epigenetic regulators included MLL2 , KDM6A and MSH6 , as well as additional mutations in SETD2 and CREBBP . KDM6A encodes for a H3K27 demethylase. We recently reported somatic KDM6A mutations in 4% of paediatric ALL at diagnosis, with mutations clustered in the catalytic jmjC domain [6] . SETD2 is the sole mammalian H3K36 trimethyltransferase, and mutations in it have been described in ETP T-ALL [2] and clear cell renal cell carcinoma [7] , but SETD2 has not been found to be recurrently mutated in large cohorts of non-ETP T-ALL [2] , [5] , [8] and AML [9] patients. MSH6 is a vital component of the DNA mismatch repair (MMR) machinery that localizes to chromatin by binding to the H3K36 trimethyl mark that SETD2 makes. SETD2 knockdown has been shown to cause mislocalization of MSH6 and microsatellite instability and a mutator phenotype in several cell types [10] . Here, we report that somatic mutations in epigenetic regulators are enriched at relapse in paediatric B-ALL with CREBBP , KDM6A , MLL2 , SETD2 and MSH6 as recurrently mutated genes. This finding suggests that therapy may be applying pressure to acquire or select for rare subclones that possess these mutations. As noted above, SETD2 and MSH6 have been linked together in DNA MMR via the H3K36 trimethyl mark. We speculate that the loss-of-function mutations identified in SETD2 and MSH6 may lead to clonal survival by at least two possible mechanisms. One, a mutator phenotype induced by SETD2 inactivation could increase the mutational diversity and thus, adaptability of the leukaemia, leading to clonal survival. Two, since intact MMR is important for triggering apoptosis and/or cell cycle arrest in response to many DNA damaging chemotherapies, SETD2 loss may lead to chemotherapy tolerance. For example, leukaemia cells lines with defective MMR show chemoresistance to the thiopurines 6-MP and 6-TG [11] , which are commonly used in ALL therapy. These mechanisms are potentially reversible by inhibiting the epigenetic regulators that oppose SETD2 activity such as the H3K36 demethylases. Interestingly, alterations in other factors which modify H3K36 methylation, such as NSD1 , WHSC1/NSD2 , NSD3 and KDM4A have been associated with ALL, AML, multiple myeloma, breast cancer and myelodysplastic syndrome [12] . Several recent reports have identified recurrent activating WHSC1 / NSD2 E1099K mutations in many ALL cell lines and 20% of ETV6-RUNX1 translocated ALL patients [13] , [14] . The genetic basis for chemoresistance and poor outcomes in relapsed ALL is beginning to be defined. For example, recent studies have identified relapse acquired NT5C2 mutations in ALL which lead to thiopurine resistance (ref 8 , 15 ). This study identifies mutations in genes encoding epigenetic regulators as frequently gained at the time of relapse. Although this study was not powered to determine a prognostic effect of these mutations in this modest cohort of patients, the enrichment of mutations in epigenetic regulators in relapsed B-ALL and other chemoresistant, high-risk subtypes of de novo leukaemia is quite suggestive of a role in clonal survival. Epigenetic regulators deserve particular attention because they are amenable to pharmacological modulation. Histone deacetylase inhibitors are currently in clinical use [16] , and histone methyltransferase inhibitors, such as DOT1L inhibitors [17] , are in clinical development. Although these epigenetic therapies are first being evaluated in the relapsed setting, our work also suggests that incorporating epigenetic therapies in upfront therapy, particularly in patients with identified mutations, could be a strategy to prevent the development of chemoresistance and relapse. Further studies are warranted to define the prognostic value of mutations in epigenetic regulators in ALL, their effects on chemotherapy resistance and whether therapeutic modulation of H3K36 methylation levels is a viable therapeutic strategy to prevent and treat relapse in patients with leukaemia. Patient materials Subjects were paediatric acute lymphoblastic patients enrolled and banked on upfront therapy protocols DFCI 00-001, DFCI 05-001, AIEOP-2000, AIEOP-2006 or Interfant-99 and their families each gave informed consent for future biological research on their banked samples under protocols approved by the Institutional Review Board at each participating institution and Dana Farber Cancer Institute. Bone marrow specimens were primarily used, but peripheral blood was used for remission samples, if no bone marrow sample was available. Diagnostic and relapse marrow samples had at least 60% blasts by morphology. Mononuclear cells from each sample were isolated with Ficoll density gradient centrifugation and genomic DNA was extracted. Exon capture For exon capture, 1–2 μg of genomic DNA was sheared with a Covaris E100 to an average size of 200 bp. Sheared DNA was end repaired, a-tailed and ligated to barcoded adaptors as per the Illumina Truseq Library Preparation protocol. Libraries were amplified with the Kapa Realtime Library Amplification kit to minimize the number of PCR cycles used (range 4–12). Library was then quantified by Kapa Realtime Quantification Kit and pooled up to six samples per lane in equimolar amounts totalling up to 500 ng of DNA. Each pool was then hybridized to a custom SureSelect In Solution Hybrid Capture RNA baitset, consisting of 19,952 baits, spanning 2.35 Mb and 472 genes ( Supplementary Table 1 ). Each capture was washed and amplified with the Kapa Realtime Library Amplification Kit and submitted for sequencing on an Illumina HiSeq 2000 100 bp single-end run. Amplicon sequencing 192 primer pairs spanning the coding regions of SETD2 , NRAS , KRAS , FLT3 , JAK2 , PTPN11 , TP53 and CDKN2A were designed and pooled into 48 primer pools and used for amplification in the Fluidigm All Access Array ( Supplementary Table 5 ). 50 ng of genomic DNA samples from 125 patients, 48 samples at a time with 48 primers pools, were amplified by the Fluidigm All Access microfluidics system and each tagged with a unique barcode. All samples were then pooled and sequenced on one Illumina Hiseq 2000 100 bp single-end run. Variant calling Fastq files were aligned to hg19 version of the human genome with BWA. SNP, indel and CNV calling was performed with samtools mpileup and Varscan 2.2.3 somatic option. Annovar was used to annotate variants. Relapsed and diagnostic variants were linked and they were filtered for ≥15% allele frequency and 20 × coverage in either tumour sample, <5% and 10 × coverage in the remission sample, bidirectional variant reads, minimal strand bias and minimal local noise. Variants were visualized in the Integrated Genome Viewer to eliminate variants with clustered read position and variants caused by indel artifacts. Sanger sequencing was used to validate a sample of somatic variants found by next generation sequencing to validate filtering criteria. Every filtered somatic variant position was then forced called on every sample to examine the baseline noisiness of each position. Those with mean baselines >1% allele frequency in remission samples were excluded. Variants were also filtered to only those positions within 50 bp of those included in the custom capture baitset. Variants were considered somatic if they were present in <5% allele frequency in the paired remission sample (to account for high minimal residual disease). How to cite this article: Mar, B. G. et al. Mutations in epigenetic regulators including SETD2 are gained during relapse in paediatric ALL. Nat. Commun. 5:3469 doi: 10.1038/ncomms4469 (2014).